Elucidating protonation pathways in CO2photoreduction using the kinetic isotope effect The surge in anthropogenic CO 2 emissions from fossil fuel dependence demands innovative solutions, such as artificial photosynthesis, to convert CO 2 into value-added products. Unraveling the CO 2 photoreduction mechanism at the molecular level is vital for developing high-performance photocatalysts. Here we show kinetic isotope effect evidence for the contested protonation pathway for CO 2 photoreduction on TiO 2 nanoparticles, which challenges the long-held assumption of electron-initiated activation. Employing isotopically labeled H 2 O/D 2 O and in-situ diffuse reflectance infrared Fourier transform spectroscopy, we observe H + /D + -protonated intermediates on TiO 2 nanoparticles and capture their inverse decay kinetic isotope effect. Our findings significantly broaden our understanding of the CO 2 uptake mechanism in semiconductor photocatalysts. The continued dependence on fossil fuels has led to a substantial increase in anthropogenic carbon dioxide (CO 2 ) emissions, culminating in deleterious environmental impacts and energy crises [1] , [2] . An optimal strategy for addressing these challenges involves the conversion of CO 2 into value-added products, such as CO and CH 4 , through artificial photosynthesis, which directly exploits incident sunlight and water [3] , [4] . However, a comprehensive understanding of the complex CO 2 photoreduction reaction at the molecular level, particularly at the CO 2 /H 2 O/catalyst gas-liquid-solid interface, remains elusive owing to the involvement of numerous proton-coupled electron transfer processes and potential reaction pathways with various intermediates [5] , [6] , [7] . Elucidating the CO 2 reduction pathway on the semiconductor catalyst surface is crucial for designing high-performance photocatalysts [8] . Upon light exposure, a comprehensive CO 2 photoreduction process typically encompasses water oxidation (or organic sacrificial agents, if utilized) and CO 2 reduction half-reactions. The water oxidation half-reaction is often regarded as analogous to the oxygen-evolving reaction (OER) in water-splitting [9] , [10] . The CO 2 reduction reaction encompasses multiple step-wise proton/electron transfer processes. Identifying the rate-determining step in such multi-step chemical reactions is an arduous task, yet essential for optimizing reaction systems. For example, the classic CO 2 + 2e − + 2H + → CO + H 2 O (−0.53 V vs. NHE) reaction on a semiconductor photocatalyst necessitates the enrichment and activation of CO 2 molecules at the gas-vapor-catalyst or gas-liquid-catalyst interface, followed by a reduction reaction through a series of fundamental steps involving consecutive proton and electron transfers [11] . As a linear non-polar molecule, CO 2 is among the most stable carbon compounds. Nevertheless, the oxygen atoms in CO 2 can donate their lone pair of electrons to surface Lewis acid centers or be protonated by Brønsted acids [12] . The carbon atom can also accept electrons from Lewis base centers, forming carbonate-like species [13] . Moreover, the π electrons of the C=O bond can interact with electron centers, leading to bond cleavage and hybridization changes from O-sp 2 to O-sp 3 . On the surface of the semiconductor catalyst, the adsorption configuration of CO 2 is also notably altered and influenced by the presence of water or other molecular proton donors [14] , [15] , [16] . All these potential reaction configurations constitute the initial steps of CO 2 activation. 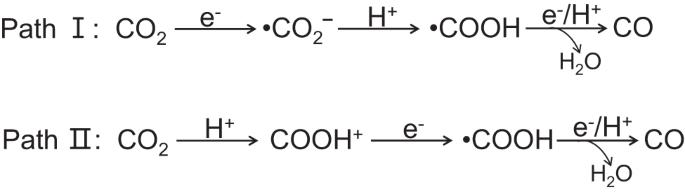Fig. 1: Initial CO2reduction mechanism. Two feasible reaction pathways for photoreduction of CO2in aqueous solution. Figure 1 illustrates two feasible reaction pathways for CO 2 photoreduction to CO in an aqueous solution: the electron-initiated pathway (path I) and the protonation pathway (path II). For a prolonged time, the initial step of CO 2 activation was presumed to occur through path I, with a negatively charged CO 2 δ•- species as the sole intermediate product [17] , [18] . However, the single-electron transfer to CO 2 is highly endergonic due to the molecule’s negative adiabatic electron affinity [19] . Additionally, the initial CO 2 uptake on hydrophilic surfaces of MO x /MS x semiconductor photocatalysts is challenging, which impedes direct single-electron transfer [20] , [21] . Instead, a protonation pathway (path II) that first polarizes CO 2 molecules, akin to the photocatalytic dehalogenation of non-polar halogenated aromatics [22] , appears more plausible. However, both pathways lack definitive, direct evidence for confirmation. Fig. 1: Initial CO 2 reduction mechanism. Two feasible reaction pathways for photoreduction of CO 2 in aqueous solution. Full size image The kinetic isotope effect (KIE) is a crucial and sensitive tool for investigating reaction mechanisms by tracking the transition state of the rate-determining step using isotopically-labeled reagents [23] , [24] . In this study, we employed isotopically labeled H 2 O/D 2 O to determine an inverse kinetic solvent isotope effect (KSIE) of 0.2~0.9 on the photoreduction of CO 2 to CO on TiO 2 nanoparticles. Our findings confirm the protonation pathway with O sp 2 −hybridized O=C=O-H + /D + intermediates (Fig. 2 ), providing the elucidation of the protonation pathway for CO 2 photoreduction and shedding light on the nature of CO 2 uptake on semiconductor photocatalysts. Fig. 2: Water-splitting and CO 2 photoreduction processes on TiO 2 . The water-splitting reaction (left) and the CO 2 photoreduction to CO (right) with isotopically labeled H 2 O/D 2 O. CPET represents concerted proton-coupled electron transfer, PT represents proton transfer, ET represents electron transfer. Full size image Inverse KIE of CO 2 photoreduction We commenced our investigation by examining the KSIE of CO 2 photoreduction to CO in a TiO 2 /water system, employing isotopically labeled H 2 O/D 2 O, and compared it to the water-splitting reaction in analogous systems (with or without CO 2 ). We first used the commercially available anatase TiO 2 (with ~20 nm-sized nanoparticles), a prevalent photocatalyst for water-splitting and CO 2 reduction, as a representative example of conventional metal oxide (MO x ) semiconductor catalysts with hydrophilic surfaces. We quantitatively detected the reduction products (i.e., H 2 , D 2 , CO) of the water-splitting and CO 2 photoreduction reactions through gas chromatography (Supplementary Fig. 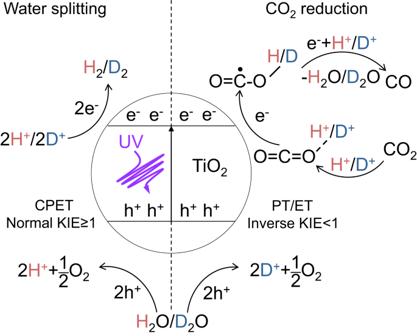Fig. 2: Water-splitting and CO2photoreduction processes on TiO2. The water-splitting reaction (left) and the CO2photoreduction to CO (right) with isotopically labeled H2O/D2O. CPET represents concerted proton-coupled electron transfer, PT represents proton transfer, ET represents electron transfer. 1 ). Control experiments conducted without CO 2 yielded negligible amounts of CO, suggesting that CO 2 reduction primarily contributes to the product formation (Supplementary Fig. 2 ). 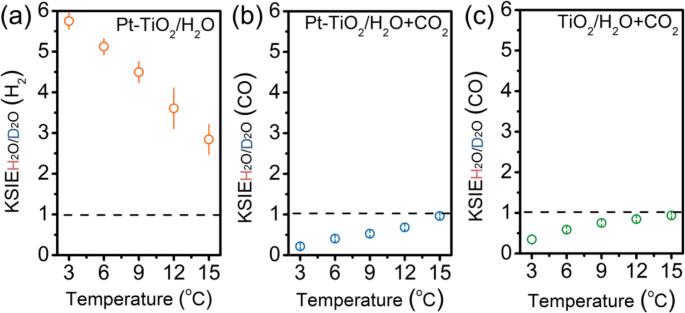Fig. 3: Comparison of kinetic solvent isotope effect (KSIE) in different reaction systems. aKSIE (H2) values obtained by comparing the H2production kinetics of the water-splitting reaction on anatase TiO2in H2O/D2O systems at different temperatures (Pt was loaded as cocatalysts, 3% chloroplatinic acid);bKSIE (CO) values obtained by comparing the kinetics of the CO2reduction reaction on anatase TiO2in H2O/D2O systems at different temperatures (Pt was loaded as cocatalysts);cKSIE (CO) values are given by comparing the CO production kinetics of the CO2reduction reaction in the H2O/D2O systems at different temperatures without Pt cocatalysts. Error bar represents three independent experiments obtaining the standard deviation. Figure 3a illustrates that H 2 production from the overall water-splitting in the Pt-TiO 2 /H 2 O system (with Pt as the hydrogen evolution reaction (HER) cocatalyst) proceeds more swiftly than with D 2 O, exhibiting a normal KSIE H2O/D2O (H 2 ) of 2.8 at 15 °C. Diminishing the reaction system’s temperature augments the KSIE value to 5.8. The same experimental phenomena could be observed regardless of whether the cocatalyst was preloaded or loaded during the reaction (Supplementary Fig. 3 ). This temperature-dependent KSIE is consistent with the primary KIE’s characteristics for O-H/O-D cleavage during the oxygen evolution reaction (OER), indicating direct O-H cleavage as the rate-determining step of water-splitting [25] , [26] , [27] . However, we observed an inverse KSIE H2O/D2O (CO) using the same catalyst in the presence of CO 2 (Fig. 3b ). As the temperature declined from 15 to 3 °C, the KSIE H2O/D2O (CO) decreased from 0.9 to 0.2. Except for adding CO 2 , all experimental conditions were congruent with the water-splitting reaction. Furthermore, the KSIE H2O/D2O (H 2 ) under identical experimental conditions displayed >1 normal values (Supplementary Fig. 4 ), suggesting different rate-determining steps between CO 2 photoreduction and water-splitting. Without Pt loading, the CO 2 photoreduction on pristine TiO 2 exhibited analogous inverse KSIE H2O/D2O (CO) values (Fig. 3c ). This outcome implies that the rate-determining step encompasses hybridization changes from sp 2 to sp 3 in the secondary inverse KIE phenomenon, consistent with the double-bond break of O=C=O molecules instead of direct O-H cleavage in OER. By employing H 2 O/D 2 O as labeled isotopes, the observed inverse KIE denotes a configuration transition between protonated intermediates O=C=O-H + /D + (O sp 2 ) and O=C • −O-H/D (O sp 3 ) during electron transfer, offering robust evidence for a protonation pathway involving the formation of the protonated intermediate O=C=O-H + as the initial step of CO 2 photoreduction (path II, Fig. 1 ). This mechanism challenges the widely accepted electron-initiated pathway (path I, Fig. 1 ). Note that such a protonation pathway does not rely on the presence of a water solvent. We introduced water in the form of vapor into the reaction instead of as a solvent, and the same inverse KIE could be observed (Supplementary Fig. 5 ). This suggests that the protonation of CO 2 can be achieved through water vapor. Fig. 3: Comparison of kinetic solvent isotope effect (KSIE) in different reaction systems. a KSIE (H 2 ) values obtained by comparing the H 2 production kinetics of the water-splitting reaction on anatase TiO 2 in H 2 O/D 2 O systems at different temperatures (Pt was loaded as cocatalysts, 3% chloroplatinic acid); b KSIE (CO) values obtained by comparing the kinetics of the CO 2 reduction reaction on anatase TiO 2 in H 2 O/D 2 O systems at different temperatures (Pt was loaded as cocatalysts); c KSIE (CO) values are given by comparing the CO production kinetics of the CO 2 reduction reaction in the H 2 O/D 2 O systems at different temperatures without Pt cocatalysts. Error bar represents three independent experiments obtaining the standard deviation. Full size image It is well-acknowledged that the characteristics of employed TiO 2 catalysts can significantly influence their interaction with target molecules and thus lead to the change in reaction kinetics. To better ascertain whether the observed KIE changes originated from the reaction pathway itself or were influenced by the catalyst material, we conducted supplementary experiments across various TiO 2 systems to bolster our findings. We first examined the influence of the TiO 2 crystal structure by comparing the KIE for the CO 2 reduction on anatase and rutile TiO 2 (characterized by XRD and TEM/HR-TEM, see Supplementary Fig. 6 and Supplementary Fig. 7 ). We found that the KSIE H2O/D2O (CO) on both anatase and rutile catalysts exhibited inverse KIE (<1), suggesting that the observed inverse KIE and the protonation pathway in CO 2 reduction are common to both crystal structures. Furthermore, we examined the effect of exposed facets of the TiO 2 catalyst. As a comparison, we synthesized anatase TiO 2 nanosheet with high exposure of the {001} facet according to a reported method [28] , which was characterized using XRD, TEM, HR-TEM, and SAED (Supplementary Fig. 8 ). The KSIE H2O/D2O (CO) for CO 2 reduction on these {001}-exposed TiO 2 nanosheets still exhibited inverse KIE < 1. These results further confirmed that the exposed facet of the TiO 2 nanoparticles does not influence the CO 2 reduction pathway under our experimental conditions. Finally, we evaluated the effect of oxygen defects. Oxygen vacancies on the TiO 2 surface are often considered active sites for the oxygen evolution reaction (OER) [29] . However, their direct influence on CO 2 reduction is less clear. We prepared oxygen-deficient TiO 2 nanoparticles according to a reported method of NaBH 4 calcination [30] , and characterized them using XRD, TEM, and ESR, which confirmed the presence of oxygen vacancies (Supplementary Fig. 9 ). The KSIE H2O/D2O (CO) for CO 2 reduction on these oxygen-deficient nanoparticles remained <1, exhibiting the secondary inverse KIE and aligning with the protonation pathway. These additional characterizations and experiments confirmed that the inverse KIE observed in the CO 2 reduction reaction is intrinsic to the TiO 2 material generalized to a broader range of TiO 2 -based photocatalytic systems, regardless of the crystal structure, exposed facet, or oxygen vacancy concentration. As a conventional metal oxide semiconductor with a hydrophilic surface and moderate reduction ability, TiO 2 demonstrates inadequate CO 2 uptake capacity [31] . As a result, the endergonic single-electron transfer of CO 2 → CO 2 δ•- on TiO 2 signifies a high-energy reaction. Nevertheless, in the photocatalytic dehalogenation of non-polar halogenated aromatics (e.g., polybrominated diphenyl ethers, PBDEs), a protonation pathway involving initial proton adhesion on the aromatic ring of PBDE molecules before subsequent electron transfer has been substantiated [22] . Additionally, in our recent work, we uncovered a step-wise proton transfer/electron transfer (PT/ET) pathway on TiO 2 for the single-electron/single-proton reduction of t Bu 3 ArO• and TEMPO• to t Bu 3 ArOH and TEMPOH [32] . These investigations support the feasibility of the protonation pathway for CO 2 photoreduction on TiO 2 catalysts. In-situ DRIFTS measurements To investigate the protonation pathway and monitor O=C=O-H + /D + intermediates during photocatalytic CO 2 reduction, we employed in-situ diffuse reflection infrared Fourier transform spectroscopy (DRIFTS) at the TiO 2 /H 2 O/CO 2 (TiO 2 /D 2 O/CO 2 ) interface. The experiment was carried out under 365 nm irradiation (3 W, LED) for 15 min, with H 2 O and CO 2 (5 mL/min) introduced into the chamber by N 2 flow (5 mL/min) until equilibrium was reached. We used the pre-reaction equilibrium system as a blank background and observed negative or positive IR signals during the reaction, indicating the loss or gain of species at the TiO 2 /H 2 O/CO 2 (TiO 2 /D 2 O/CO 2 ) interface. Control experiments demonstrated that in the absence of incident light, the reaction did not occur (Supplementary Fig. 10 ). 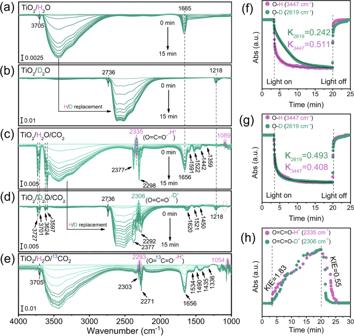Fig. 4: In-situ diffuse reflectance infrared Fourier transform spectroscopy (DRIFTS) measurements. DRIFTS spectra collected at the TiO2/H2O (a), TiO2/D2O (b), TiO2/H2O/CO2(c), TiO2/D2O/CO2(d) and TiO2/H2O/13CO2(e) interfaces under constant 365 nm (3 W, LED) irradiation in 15 min;fTime profiles of IR signals at 3447 cm−1in (a) and 2619 cm−1in (b) from light-on to light-off, representing the decay kinetics of O-H and O-D in water-splitting;gTime profiles of IR signals at 3447 cm−1in (c) and 2619 cm−1in (d) from light-on to light-off, representing the decay kinetics of O-H and O-D in CO2photoreduction;hTime profiles of IR signals at 2335 cm−1and 2306 cm−1(after baseline corrections to maintain positive values) from light-on to light-off, representing the formation and decay kinetics of O=C=O-H+and O=C=O-D+. An inverse KIE was obtained during the decay process after light-off. Pink shading represents the peak position of the COOH+intermediate, and green shading represents the peak position of the COOD+intermediate. 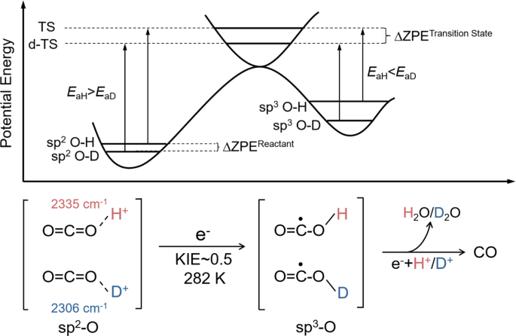Fig. 5:The source of inverse KIE. Schematic illustrations and energetic profiles of the O=C=O-H+/D+→ O=C•−O-H/D electron transfer process. TS represents transition state, ZPE represents zero-point energy. Figure 4a reveals negative peaks at 3700–2800 cm −1 and 1665 cm −1 at the TiO 2 /H 2 O interface upon constant irradiation, corresponding to the O-H stretching and H-O-H bending vibrations of H 2 O molecules [33] , respectively. The weak signal at 3705 cm −1 represented the terminal O-H group on the TiO 2 surface [34] . When H 2 O was replaced with D 2 O, noticeable redshifts of both O-D stretching and D-O-D bending vibrations to 2700–2100 cm −1 and 1218 cm −1 were observed (Fig. 4b ), in line with the theoretical H/D replacement effect [35] , [36] . The decay kinetics of O-H/O-D stretching vibrations showed that the O-H signal decays much faster than the O-D signal, resulting in a direct KIE of 2.11 (Fig. 4e ), consistent with the measured normal KSIE H2O/D2O (H 2 ) values and representing features of the direct O-H/-D cleavage during overall water-splitting. Fig. 4: In-situ diffuse reflectance infrared Fourier transform spectroscopy (DRIFTS) measurements. DRIFTS spectra collected at the TiO 2 /H 2 O ( a ), TiO 2 /D 2 O ( b ), TiO 2 /H 2 O/CO 2 ( c ), TiO 2 /D 2 O/CO 2 ( d ) and TiO 2 /H 2 O/ 13 CO 2 ( e ) interfaces under constant 365 nm (3 W, LED) irradiation in 15 min; f Time profiles of IR signals at 3447 cm −1 in ( a ) and 2619 cm −1 in ( b ) from light-on to light-off, representing the decay kinetics of O-H and O-D in water-splitting; g Time profiles of IR signals at 3447 cm −1 in ( c ) and 2619 cm −1 in ( d ) from light-on to light-off, representing the decay kinetics of O-H and O-D in CO 2 photoreduction; h Time profiles of IR signals at 2335 cm −1 and 2306 cm −1 (after baseline corrections to maintain positive values) from light-on to light-off, representing the formation and decay kinetics of O=C=O-H + and O=C=O-D + . An inverse KIE was obtained during the decay process after light-off. Pink shading represents the peak position of the COOH + intermediate, and green shading represents the peak position of the COOD + intermediate. Full size image In the TiO 2 /H 2 O/CO 2 system (Fig. 4c ), negative peaks at 2377 cm −1 and 2298 cm −1 corresponding to the C=O stretching vibrations of CO 2 were observed, along with an emerging positive signal peak at 2335 cm −1 adjacent to the decayed stretching vibration signals of CO 2 , likely due to the formation of the protonated CO 2 intermediate (O=C=O-H + ). The adhesion of a proton to the oxygen atom would alter the C=O bond and alter the effective mass of oxygen, thereby changing the vibration frequency. In addition, according to Hooke’s Law, the adhesion of protons to the oxygen nucleus in C=O bonds increases the effective mass of the oxygen atom, which subsequently results in a change in the frequency of the stretching vibrations of the C=O bond [37] . Moreover, the increasing positive signal at 1089 cm −1 is likely from the C=O-H + bending vibration. Negative peaks at 3727 cm −1 , 3701 cm −1 , 3624 cm −1 , and 3597 cm −1 corresponded to the weak overtone region of CO 2 molecules [38] , and signals at 1591 cm −1 , 1522 cm −1 , 1442 cm −1 , and 1359 cm −1 were assigned to -COOH* species, monodentate carbonate (m-CO 2-3 ) groups, as well as the antisymmetric and symmetric stretching bands of bidentate carbonate (b-CO 2-3 ) groups [39] , [40] , respectively. To verify that the observed changes in CO 2 FT-IR signals resulted from a surface reaction rather than a modification in the surface adsorption configuration of CO 2 under incident light, we carried out a control experiment. This involved first running the reaction for a specified time under light, followed by the removal of the gas phase using a N 2 flow. By subtracting the equilibrium background in N 2 prior to the experiment, we were able to observe changes in surface-adsorbed species over time. Given that the removal of the CO 2 gas phase would cut off the replenishment of surface CO 2 , a fading CO 2 signal would suggest that the observed signals stemmed from the reaction rather than adsorption. Otherwise, we would observe unchanged, stable adsorbate signals. As illustrated in Supplementary Fig. 11c, d , after the abrupt removal of CO 2 , both the negative and positive signals of C=O vibration from CO 2 species around 2330 cm −1 to 2340 cm −1 continued to decrease over time and vanished within tens of seconds. This suggests that the observed CO 2 signals are not from a stable adsorbate but from a surface reaction. Furthermore, to validate the assignment of the protonated O=C=O-H + intermediate, we replaced H 2 O with deuterated-labeled D 2 O under identical conditions. The diagnostic signal peak of the protonated intermediate shifted towards a lower wavenumber from 2335 cm −1 to 2306 cm −1 upon replacing O=C=O-H + with O=C=O-D + (Fig. 4d ). The negative signal peaks (both stretching bands and overtone region) of CO 2 molecules remained unchanged. This H/D replacement effect on the C=O stretching vibration of O=C=O-H + /D + intermediates is consistent with the results of Hooke’s Law (detailed calculation formula see supplementary methods). However, the C=O-D + bending vibration was not observed in O=C=O-D + , which likely shifts a lower frequency, beyond our in-situ DRIFTS detection range (Fig. 4d ). Together with the H/D replacement experiments without CO 2 , the shift of the diagnostic peak of O=C=O-D + compared to that of the unlabeled O=C=O-H + provides direct evidence for the formation of protonated O=C=O-H + intermediates during the CO 2 photoreduction process at the TiO 2 /H 2 O/CO 2 interface. Furthermore, we have an additional DRIFTS experiment using 13 C-labeled 13 CO 2 . As depicted in Fig. 4e , a distinct redshift from 2335 cm −1 to 2293 cm −1 of the C=O stretching vibration was observed when employing 13 CO 2 , corresponding to the shift of the 13 C=O stretching vibration signal in O= 13 C=O-H + compared to the unlabeled 12 C=O in O=C=O-H + /D + (2335 cm −1 /2306 cm −1 ) due to the 12 C/ 13 C isotope replacement effect. Moreover, the bending vibration of C=O-H + at 1089 cm −1 was also shifted to 1054 cm −1 in the 13 CO 2 system corresponding to 13 C=O-H + . These findings are highly consistent with our KIE experimental results and further validates our assignment. Quantum chemical calculations We further conducted quantum chemical calculations to simulate the infrared signals of the H + /D + protons adhered to the oxygen atom in CO 2 . The results are consistent with our assumption that the C=O stretching vibration in CO 2 does not form a C-O-H sp 3 structure after adhering to a H + /D + proton, thereby a C-O signal does not appear (Supplementary Fig. 12 ). It remains at 2300–2400 cm −1 (the discrepancy between the calculation and actual data should come from different adsorption interfaces; the calculation only simulates the situation in a vacuum). The vibration frequency changes from protonated species and pristine CO 2 due to the influence of bond energy and the effective mass of oxygen. Moreover, replacing H + with D + indeed causes the simulated C=O stretching vibration to shift to a lower frequency (2403 cm −1 → 2394 cm −1 ). Interestingly, quantum calculations also reveal possible O-H/O-D stretching vibrations (3406 cm −1 /2490 cm −1 ), which are not clearly observed in the actual experiment due to the significant influence of water signals. More importantly, we found that the 960 cm −1 in O=C=O-H + corresponds to the bending vibration of C=O-H + , which correspond to the positive signal at 1089 cm −1 observed in in-situ DRIFTS. In O=C=O-D + , the bending vibration of C=O-D + shifts to a lower frequency, beyond our in-situ DRIFTS detection range, fully consistent with our observation. However, when 13 C is used for simulation, the bending vibration of 13 C=O-H + can be seen to shift from 960 cm −1 to 952 cm −1 . In our actual in-situ DRIFTS, when using 13 CO 2 , we indeed observed a shift towards a lower wavenumber of the 13 C=O-H+ bending vibration (1054 cm −1 ) from C=O-H + (1089 cm −1 ) using unlabeled CO 2 (Fig. 4e ). This result fully support our assignment of the O=C=O-H + signal. In prior research, the generation of CO 2 δ•- anion radicals have been detected during the photocatalytic degradation of formate on TiO 2 nanoparticles using infrared (IR) and electron spin resonance (ESR) spectroscopy [41] , [42] . Although the CO 2 δ•- anion radical is often cited as the exclusive intermediate of the initial step in CO 2 photoreduction, no definitive evidence has been provided for its presence in CO 2 photoreduction systems. On a polar TiO 2 surface surrounded by H 2 O molecules, chemisorbed species, mainly OH − , produce distinct π or δ resonances, while physisorbed species have weak signals [43] . This limits the opportunities for single-electron transfer by neutral physisorbed CO 2 molecules, which are scarce at the polar H 2 O/TiO 2 interface. Instead, an ionized CO 2 moiety promotes interfacial CO 2 uptake [44] , facilitating subsequent electron/proton transfer. Under our experimental conditions, the only visible positive signal peak after light illumination corresponds to the protonated O=C=O-H + /D + signal. This finding contradicts previous understandings of the CO 2 photoreduction mechanism and suggests a protonation pathway [45] . We also compared the decay kinetics of O=C=O-H + /D + and O-H/O-D during the reaction. The inverse kinetic isotope effect (KIE) of the O sp 2 → O sp 3 hybrid transition process is a classic phenomenon in reaction kinetics associated with the disparity in the vibration frequency of chemical bonds [22] , [46] . The observed inverse KIE of O=C=O-H + /D + decay (KIE = 0.55) provides strong evidence for the protonation pathway (Fig. 4h ; Supplementary Fig. 13 ), which involves the O=C=O-H + /D + → O=C • −O-H/D double-bond break with a hybridization change from O sp 2 → O sp 3 via additional electron transfer (Fig. 5 ). In most reactions, the overall rate is determined by the slowest step, known as the rate-determining step [47] . In our system, without CO 2 , the direct breakage of the O-H/O-D bond undeniably constitutes the rate-determining step, hence its KIE is greater than 1 (Fig. 4f ). However, the decay kinetics of O-H/O-D stretching vibration also exhibited an inverse KIE = 0.827 in the presence of CO 2 (Fig. 4g ), indicating that the slower reduction reaction of CO 2 (in this case, the reduction of the protonated intermediate) becomes the rate-determining step. Fig. 5: The source of inverse KIE . Schematic illustrations and energetic profiles of the O=C=O-H + /D + → O=C • −O-H/D electron transfer process. TS represents transition state, ZPE represents zero-point energy. Full size image In this study, we unveil a mechanism governing the photoreduction of CO 2 on semiconductor catalysts, which transpires via a protonation pathway. We report the formation of an O=C=O-H + intermediate, which exhibits an inverse KIE during the subsequent electron transfer process. This electron transfer process prompts the conversion of the sp 2 −hybridized O=C=O-H + /D + species into the sp 3 −hybridized O=C • −O-H/D species. Utilizing isotopically labeled in-situ DRIFTS, we successfully discern the formation of H + /D + -protonated O=C=O-H + /D + intermediates on TiO 2 nanoparticles and capture their inverse decay KIE. This research substantially broadens our comprehension of the CO 2 uptake mechanism in semiconductor photocatalysts, necessitating a re-examination of long-held assumptions within the field. Our findings hold significant potential for advancing the development of more efficient and sustainable photocatalytic CO 2 reduction technologies in the future. Materials Commercial titanium dioxide (TiO 2 , anatase, 20 nm), sodium borohydride (NaBH 4 ), tetrabutyl titanate, hydrofluoric acid (HF, 40 wt%), chloroplatinic acid (H 2 PtCl 6 ·6H 2 O), ethanol and deuterium oxide (D 2 O, 99.9 atom % D) were purchased from Shanghai McLean Biochemical Technology Co., Ltd. All reagents used in the synthesis were analytically pure and had not been further purified. Deionized water was obtained from a purified distillation unit in the laboratory. Before any photocatalytic reaction experiments, TiO 2 samples were first calcinated and then illuminated by an ultraviolet lamp (365 nm, 160 mW∙cm −2 ) in water. Synthesis of (001) exposed TiO 2 nanosheet In a typical synthesis, 12.5 mL of tetrabutyl titanate was mixed with 2 mL of HF solution, under stirring for 30 min. The solution was then transferred into a 50-mL Teflon-lined autoclave, and kept at 180 °C for 24 h. After the solvothermal reaction, the resulting white precipitates were collected and washed with ethanol and distilled water for three times. The samples were dried in a vacuum oven at 60 °C for 12 h. Synthesis of oxygen-deficient TiO 2 1 g TiO 2 nanoparticle powder was mixed with 2 g NaBH 4 and the mixture was ground for 30 min thoroughly. Then the mixture was transferred into a porcelain boat, and placed in a tubular furnace, heated from room temperature to 350 °C/1 h under an Ar atmosphere at a heating rate of 10 °C min −1 . After naturally cooling down to room temperature, the colored TiO 2 was obtained, simply washed with deionized water and ethanol several times to remove unreacted NaBH 4 , and dried at 70 °C. Water-splitting experiments In a typical procedure, 50 mg TiO 2 powder was dispersed in 10 mL deionized water (H 2 O) and 10 mL deuterium water (D 2 O), respectively. Next, 3 wt% Pt as cocatalysts was loaded via in-situ photo deposition using H 2 PtCl 6 ·6H 2 O without any sacrificial agents. After irradiation with an ultraviolet lamp (365 nm, 160 mW∙cm −2 ), Gas products were determined by using a gas chromatography (GC-7900) equipped with the TCD thermal conductivity detector and the carrier gas was chosen Ar. CO 2 photoreduction experiments CO 2 photoreduction was carried out in a sealed self-made 150 mL stainless-steel reactor with an ultraviolet lamp (365 nm, 160 mW∙cm −2 ) as the light source. In a typical procedure, 50 mg catalyst was dispersed in 10 mL deionized water (H 2 O) and 10 mL deuterium water (D 2 O), respectively. CO 2 was then introduced into the reactor and bubbled for 25 min to completely remove air. Gas products were detected by the gas chromatography (GC-7920, China) equipped with hydrogen flame ionization detector (FID) and thermal conductivity detector (TCD). In addition, the control experiment had the same experimental conditions as described above except for the addition of 3 wt% Pt as cocatalysts; In the gas-solid reaction system, 50 mg catalyst was dispersed in quartz grooves, add 2 ml of water or deuterated water to the bottom of the 150 ml reactor with no direct contact with the catalyst, assuring that water participates in the reaction in vapor state. CO 2 flow was then introduced into the reactor for 25 min before light-on. In-situ DRIFTS experiments In-situ diffuse reflection infrared Fourier transform spectroscopy (DRIFTS) experiments were conducted on a Nicolet iS10 (Thermo) machine according to our previous work [47] . In a typical procedure, catalyst sample was sealed in the reaction chamber with a quartz window. CO 2 and H 2 O (or D 2 O) were carried into the reaction chamber by N 2 flow until equilibrium. After taking the equilibrium system before reaction as the blank background, IR signals were collected in-situ during the incident irradiation of a 365 nm LED lamb (3 W) through the quartz glass window. Hooke’s law Taking diatomic as an example, when the diatomic is telescopic and vibrating, they can be approximated as a simple harmonic oscillator. Given two bodies, one with mass m 1 and the other with mass m 2 , the equivalent one-body problem, with the position of one body with respect to the other as the unknown, is that of a single body of mass; where the equivalent mass of O=C=O-H + is m 1 = 12 (C), m 2 = 17 (O-H, v 1 = 2335 cm −1 ); The equivalent mass of O=C=O-D + is m 1 = 12 (C), m 2 = 18 (O-D, v 2 = 2306 cm −1 ). Composite  mass:μ=1/1/m_1+1/m_2=m_1m_2/m_1+m_2
 (1) 
    Vibration  frequency:υ=1/2π√(k/μ)
 (2) When v 1 = 2335 cm −1 : The force constants of chemical bonds: 
    k=μ(2πυ_1)^2=m_1m_2/m_1+m_2(2πυ_1)^2=12× 17/12+17(2× 3.14× 2335)^2=1.51×10^9
 When the equivalent mass of O=C=O-D + is m 1 = 12, m 2 = 18: 
    υ_2=1/2π√(k/μ)=1/2π√(k/m_1m_2/m_1+m_2=)1/2× 3.14√(1.51×10^9/12× 18/12+18=2308)